Functional and molecular features of the calmodulin-interacting protein IQCG required for haematopoiesis in zebrafish We previously reported a fusion protein NUP98–IQCG in an acute leukaemia, which functions as an aberrant regulator of transcriptional expression, yet the structure and function of IQCG have not been characterized. Here we use zebrafish to investigate the role of iqcg in haematopoietic development, and find that the numbers of haematopoietic stem cells and multilineage-differentiated cells are reduced in iqcg -deficient embryos. Mechanistically, IQCG binds to calmodulin (CaM) and acts as a molecule upstream of CaM-dependent kinase IV (CaMKIV). Crystal structures of complexes between CaM and IQ domain of IQCG reveal dual CaM-binding footprints in this motif, and provide a structural basis for a higher CaM–IQCG affinity when deprived of calcium. The results collectively allow us to understand IQCG-mediated calcium signalling in haematopoiesis, and propose a model in which IQCG stores CaM at low cytoplasmic calcium concentrations, and releases CaM to activate CaMKIV when calcium level rises. Chromosomal translocations have been shown to have an essential role in tumorigenesis, particularly in human leukaemias. In acute leukaemia, chromosomal translocations can lead to either deregulated expression of oncogenes or formation of fusion genes. Numerous studies demonstrated that genes involved in these fusions are functionally important, in that they encode transcription factors, signalling proteins or other key molecules associated with the regulation of normal development and cell proliferation, differentiation and survival, particularly in the context of haematopoiesis. Interestingly, the gene encoding nucleoporin 98 kDa ( NUP98 ), a member of nucleoporin family of nuclear pore complex components [1] , has so far been reported to fuse with at least 30 partner genes in acute leukaemia involving 11p15 translocation [2] , [3] , [4] , [5] , [6] . Two major categories of genes have been identified as fusion partners of NUP98 : genes encoding the homeobox transcription factors and those encoding non-homeobox partners, including both nuclear and cytoplasmic proteins. IQCG is a gene that we previously cloned from an acute T-lymphoid/myeloid leukaemia with a complex chromosomal translocation t(3;11)(q29q13;p15)del(3)(q29), which resulted in a fusion gene NUP98–IQCG [7] . The resultant NUP98–IQCG fusion protein behaved as an aberrant nuclear protein disturbing transcriptional expression, stimulating proliferation and partially blocking differentiation of haematopoietic stem/progenitor cells. Recently, we demonstrated that NUP98–IQCG alone could initiate an acute myeloid leukaemia in a retrovirus-transduced murine bone marrow transplantation system (Zhang et al ., personal communication), implying that the IQCG moiety in the fusion protein could exert effects on major cellular regulatory network. However, the role of the wild-type (WT) IQCG remains elusive. Hence, characterization of the functional and structural features of IQCG should not only reveal its associated pathways in physiological processes, but also shed light on the leukaemogenic mechanism of NUP98–IQCG. Sequence analyses predict two functional domains in the IQCG protein: a central coiled-coil domain and a C-terminal IQ (isoleucine–glutamine) motif ([I,L,V]QxxxR[G,x]xxx[R,K] in sequence, where x stands for any amino-acid residue) that has been shown to interact with calmodulin (CaM) in a calcium-independent manner. IQ motif-containing molecules include well-studied members ranging from myosins to voltage-operated ion channels [8] . Some IQ motif-containing proteins such as neuromodulin and neurogranin have been proposed to function as local stores of CaM [9] , [10] . The above information provided us with important clues that IQCG could have a functional link to calcium signalling. On the other hand, as zebrafish has emerged as an important model organism for studying haematopoiesis and related diseases, we used zebrafish to study the role of IQCG at the organism level. It has been well established that the highly conserved CaM represents the major calcium ion (Ca 2+ ) sensor in eukaryotic cells. It comprises two globular domains, termed N-terminal and C-terminal lobes (N- and C-lobes), connected by a flexible tether sequence [11] . Each lobe contains a pair of EF hand motifs, which are topologically helix-loop-helix domains coordinating Ca 2+ binding within their loop region [12] . Structurally, CaM assumes large conformational changes upon Ca 2+ binding, exposing hydrophobic surfaces buried within each lobe (from Ca 2+ -unbound closed conformation to Ca 2+ -bound open conformation [13] ) in favour of its interaction with target peptide sequences that usually have a propensity to form a basic amphiphilic α-helix [14] , [15] , [16] . Among the targets of CaM are members of the CaM-dependent kinase (CaMK) family, such as CaMKI and CaMKII that are expressed ubiquitously, while CaMKIV is found predominately in neuronal and haematopoietic tissues [17] , [18] . A previous study showed that CaMKIV is implicated in haematopoietic stem cell (HSC) maintenance: murine CaMKIV −/− c-Kit + Sca1 + Lin −/low cells (KSL cells) are reduced in number and unable to reconstitute blood cells upon serial transplantation [17] . Mechanistically, Ca 2+ -bound CaM activates CaMKIV by releasing the kinase’s autoinhibitory region that otherwise masks a key phosphorylation site [19] . In the present work, we identified a functional role of iqcg in the CaM-mediated calcium signalling pathway in zebrafish haematopoietic development. Our results indicate that zebrafish Iqcg serves as a regulator in definitive haematopoiesis and acts upstream of CaMKIV. Furthermore, we determine the crystal structures of IQCG IQ motif in complex with CaM that allow us to propose a model of IQCG-modulated activity of CaMKIV. Characterization of the zebrafish iqcg orthologue A search in the zebrafish genome revealed a unique orthologue of the human IQCG gene. The zebrafish iqcg gene encodes a protein of 346 amino-acid residues that exhibits 39% and 36% identity to its mouse and human orthologues, respectively. IQCG proteins, from zebrafish to human, contain tandem coiled-coil domains and an IQ motif ( Supplementary Fig. 1a ), of which the IQ motif is highly conserved ( Supplementary Fig. 1b ). As shown in Supplementary Fig. 1c , PCYT1A , LRCH3 , IQCG and RPL35A define an ~2-Mb genomic region on human chromosome 3, which is syntenic to the zebrafish iqcg genomic locus on chromosome 18. To examine the spatial and temporal expression of iqcg during embryogenesis, whole-mount mRNA in situ hybridization (WISH) assays were performed using digoxigenin-labelled antisense RNA probe. As shown in Supplementary Fig. 1d , strong signals were detectable in the blastomeres of the one and two-cell stages, indicating that iqcg transcripts were maternally derived and suggesting a role in early embryonic development ( Supplementary Fig. 1d ). After 24 h post fertilization (h.p.f. ), iqcg transcripts were detected throughout the entire embryo, predominantly expressed in brain and pronephric ducts ( Supplementary Fig. 1d ). In adult zebrafish, iqcg expression mainly localized to testis, followed by brain, kidney and ovary, while its expression was reduced in heart, liver, gut and intestine ( Supplementary Fig. 1e ). The iqcg expression pattern in zebrafish is similar with that in human tissues [7] and mice ( Supplementary Fig. 1f ). Taken together, these results indicate that zebrafish iqcg is an evolutionarily conserved orthologue of human IQCG . It is both maternally and zygotically expressed throughout early development and highly enriched in adult zebrafish kidney, the haematopoietic organ. Knockdown of iqcg depletes definitive haematopoiesis We then investigated the function of iqcg during zebrafish haematopoiesis in the developing zebrafish larvae using its specific morpholino oligonucleotides (MOs). Two antisense MOs were designed to block the translation of iqcg mRNA, whereas a morpholino with five mismatched nucleotides (denoted as 5 mm) was used as a control. MO1 targets a sequence spanning the translation start codon, whereas MO2 covers part of the 5′ untranslated region of iqcg ( Supplementary Fig. 1a ). Enhanced green fluorescent protein ( EGFP ) mRNA reporter containing MO-targeting sequences were co-injected with MOs into one-cell stage embryos to test the efficiency of these morpholinos. The results indicated that both MO1 and MO2 were able to efficiently and specifically block the translation of the EGFP reporter ( Supplementary Fig. 1g–j ). Zebrafish has primitive and definitive waves of haematopoiesis that closely resembles haematopoietic development in mammals. Its primitive haematopoietic cells appear intra-embryonically in two locations called the intermediate cell mass and the anterior lateral mesoderm [20] . To examine the primitive haematopoiesis in iqcg morphants, expression levels of some key primitive haematopoietic genes in the intermediate cell mass and the anterior lateral mesoderm regions were visualized by WISH. The results showed that expression levels of scl (for HSCs), pu.1 and gata1 (for myeloid and erythroid progenitors, respectively), and α-E1 (for haemoglobin of mature red cells) were all unaffected ( Supplementary Fig. 1k–n ). Therefore, iqcg is not likely to be involved in the zebrafish primitive haematopoiesis. We next looked at the definitive haematopoiesis. Definitive HSCs emerge directly from the ventral wall of the dorsal aorta within the aorta-gonad-mesonephros (AGM) [21] , [22] , [23] , and subsequently migrate through the blood to the caudal haematopoietic tissue (CHT), which is equivalent to the mammalian fetal liver [24] . Then, the definitive HSCs differentiate, expand and further migrate to seed the kidney and thymus, of which the former is comparable to the bone marrow of mammals; the latter is a site of lymphocyte maturation. Severe reduction of the CHT could be observed as 72 h.p.f. in iqcg morphants. The distances between caudal aorta (ca) and cardinal vein (cv) in these animals were much shorter than control embryos ( Fig. 1a ). In contrast, the ca, cv and intersomitic vessels were intact, as shown by the blood vessel endothelium marker flk1 ( Fig. 1b ). As the CHT is an essential tissue in definitive haematopoiesis [24] , [25] , we examined whether the definitive HSC were impaired in iqcg morphants. C-myb , a marker for HSC and myeloid progenitor cells, was severely reduced in the CHT of iqcg morpholino-injected embryos compared with controls at 48 h.p.f. ( Fig. 1c ). Furthermore, we found that the number of c-myb:eGFP + cells was significantly lower in iqcg morphants in the CHT at 36 h.p.f., which suggested a reduced c-myb -positive cell number ( Fig. 1d and Supplementary Fig. 2a ). As MO1 and MO2 produced similar phenotypes, we used MO1 to carry out further studies. 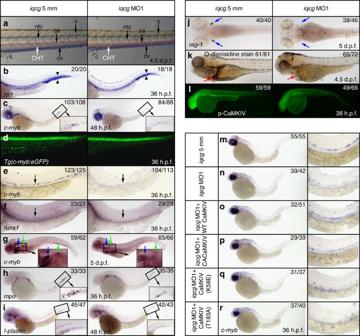Figure 1:Iqcgmorphants show deficient definitive haematopoiesis and reactivation of CaMKIV rescues thec-mybexpression. (a)Iqcgmorphants show disordered CHTs, diminished HSC population and multilineage haematopoiesis. Tails at 4.5 d.p.f. were analysed with control (5 mm for five mismatched nucleotides) and test (MO1) morpholinos. The red and blue lines were drawn to indicate the site of ca and cv, respectively. (b) Whole-mount mRNAin situhybridization (WISH) offlk1expression in controls andiqcgmorphants at 36 h.p.f. (c) WISH ofc-mybexpression in controls andiqcgmorphants at 48 h.p.f. (d) The CHT regions ofTg(c-myb:eGFP)injected withiqcgMO1 oriqcg5 mm MO were analysed. (e–j) WISH of HSC or multilineage markers in controls andiqcgmorphants. (k) O-dianisidine staining of haemoglobin in controls andiqcgmorphants at 5 d.p.f. (l) Whole-mount immunofluorescence of p-CaMKIV in controls andiqcgmorphants at 36 h.p.f. Anatomical landmarks: caudal haematopoietic tissue (CHT), caudal aorta (ca), cardinal vein (cv), cloaca (c), notochord (ntc) and somite muscles (s). The blue, green and red arrows indicate the thymus, kidney and heart, respectively. All the left panels are control embryos, whereas all the right panels areiqcgmorphants. (m–r) Reactivation of CaMKIV rescues thec-mybexpression iniqcgmorphants. Rescue experiments within vitrosynthesized WT CaMKIV (o), CACaMKIV (p), DNCaMKIV (K58E) (q) or DNCaMKIV (T183A) (r) mRNAs. WISH ofc-mybexpression in the indicated embryos at 36 h.p.f. Right panels are enlarged views of the AGM regions corresponding to the left panels. Figure 1: Iqcg morphants show deficient definitive haematopoiesis and reactivation of CaMKIV rescues the c-myb expression. ( a ) Iqcg morphants show disordered CHTs, diminished HSC population and multilineage haematopoiesis. Tails at 4.5 d.p.f. were analysed with control (5 mm for five mismatched nucleotides) and test (MO1) morpholinos. The red and blue lines were drawn to indicate the site of ca and cv, respectively. ( b ) Whole-mount mRNA in situ hybridization (WISH) of flk1 expression in controls and iqcg morphants at 36 h.p.f. ( c ) WISH of c-myb expression in controls and iqcg morphants at 48 h.p.f. ( d ) The CHT regions of Tg(c-myb:eGFP) injected with iqcg MO1 or iqcg 5 mm MO were analysed. ( e – j ) WISH of HSC or multilineage markers in controls and iqcg morphants. ( k ) O-dianisidine staining of haemoglobin in controls and iqcg morphants at 5 d.p.f. ( l ) Whole-mount immunofluorescence of p-CaMKIV in controls and iqcg morphants at 36 h.p.f. Anatomical landmarks: caudal haematopoietic tissue (CHT), caudal aorta (ca), cardinal vein (cv), cloaca (c), notochord (ntc) and somite muscles (s). The blue, green and red arrows indicate the thymus, kidney and heart, respectively. All the left panels are control embryos, whereas all the right panels are iqcg morphants. ( m – r ) Reactivation of CaMKIV rescues the c-myb expression in iqcg morphants. Rescue experiments with in vitro synthesized WT CaMKIV ( o ), CACaMKIV ( p ), DNCaMKIV (K58E) ( q ) or DNCaMKIV (T183A) ( r ) mRNAs. WISH of c-myb expression in the indicated embryos at 36 h.p.f. Right panels are enlarged views of the AGM regions corresponding to the left panels. Full size image Given that zebrafish has several haematopoietic sites, we examined the c-myb expression in the AGM, kidney and thymus. Upon MO knockdown of iqcg , the transcription levels of c-myb and another HSC marker, runx1 , in the AGM region were reduced ( Fig. 1e,f ). At 5 days post fertilization (d.p.f. ), c-myb + cells were abolished in the haematopoietic organs, that is, kidney and thymus, in iqcg morphants ( Fig. 1g ). These data indicate that loss of iqcg expression depletes definitive HSCs. We subsequently investigated the differentiated haematopoietic cells in iqcg morphants. Indeed, the expression levels of gene markers for neutrophils (that is, mpo ), monocytes and macrophages (that is, l-plastin ) as well as lymphoblasts (that is, rag1 ) were all severely impaired ( Fig. 1h–j ), indicating a decrease of these specific cell types. Furthermore, O-dianisidine staining showed very weak haemoglobin level in the iqcg morphants ( Fig. 1k ) at 4.5 d.p.f., while in control embryos the heart was filled with erythrocytes, suggesting decreased erythropoiesis in the iqcg morphants. IQCG is a CaM-binding protein We then tried to explore the molecular mechanisms governing the critical role of IQCG in haematopoiesis. IQCG molecule possesses a putative IQ motif that is believed to bind CaM in a Ca 2+ -independent fashion [8] ( Supplementary Fig. 1a ). To experimentally verify the interactions between IQCG proteins and CaM, we first performed co-immunoprecipitation (Co-IP) assays. Both human IQCG (Hs_IQCG) and zebrafish Iqcg (Dr_Iqcg) precipitated CaM when calcium was chelated by EGTA ( Fig. 2a ). In contrast, IQCG proteins lacking their IQ motifs (residues 392–419 for Hs_IQCG and residues 302–324 for Dr_Iqcg) did not precipitate CaM efficiently under the same conditions ( Fig. 2b ). We therefore conclude that IQCG proteins indeed interact with CaM, and the interactions critically depend on the IQ motifs. 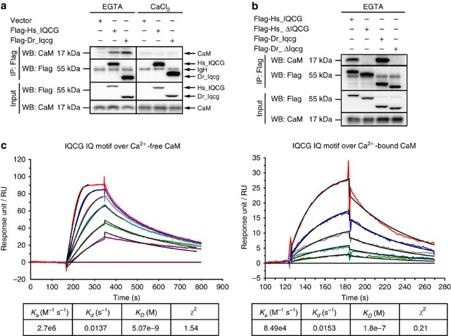Figure 2: IQCG interacts with CaM mediated by the IQ motif. (a) Ability of Hs_IQCG and Dr_Iqcg to interact with CaM, as determined by Co-IP experiments. Anti-Flag M2 affinity gel was used for immunoprecipitation (IP); antibodies to CaM or Flag were used for western blot (WB). (b) The IQ motif is required for the interaction of IQCG with CaM. ΔIQCG refers to the IQCG construction with IQ motif deleted. (c) SPR-binding experiments of human IQ motif over immobilized CaM in Ca2+-free (left panel) or Ca2+-supplemented condition (right panel). The concentrations of IQCG IQ motif were 8.4–50 nM and 20–320 nM, respectively. The curves represent direct fits of the 1:1 Langmuir-binding model to the data. Figure 2: IQCG interacts with CaM mediated by the IQ motif. ( a ) Ability of Hs_IQCG and Dr_Iqcg to interact with CaM, as determined by Co-IP experiments. Anti-Flag M2 affinity gel was used for immunoprecipitation (IP); antibodies to CaM or Flag were used for western blot (WB). ( b ) The IQ motif is required for the interaction of IQCG with CaM. ΔIQCG refers to the IQCG construction with IQ motif deleted. ( c ) SPR-binding experiments of human IQ motif over immobilized CaM in Ca 2+ -free (left panel) or Ca 2+ -supplemented condition (right panel). The concentrations of IQCG IQ motif were 8.4–50 nM and 20–320 nM, respectively. The curves represent direct fits of the 1:1 Langmuir-binding model to the data. Full size image To assess if the binding between CaM and IQCG is direct, the IQ motif of human IQCG (residues 389–423) was purified as the analyte to perform surface plasmon resonance (SPR)-binding experiments for measuring binding affinities to CaM. The IQCG-binding experiments were carried out with GST-CaM in buffer containing EDTA or CaCl 2 . The SPR-binding curves are shown in Fig. 2c for Ca 2+ -free CaM (left panel) and Ca 2+ -bound CaM (right panel), respectively. The association rates ( K a or K on ) showed substantial differences, whereas dissociation rates ( K d or K off ) kept similar between these two conditions. Based on the binding kinetics, the equilibrium dissociation constants ( K D ) were calculated. The K D for IQ motif of human IQCG (residues 389–423) with Ca 2+ -free CaM was 5.07 nM, whereas K D with Ca 2+ -bound CaM was 180 nM, which meant that IQCG binding to Ca 2+ -free CaM is ~45 fold stronger than that to Ca 2+ -bound CaM. The SPR results are consistent with the Co-IP results, and confirm that IQCG is a CaM-binding protein. CaMKIV acts downstream of IQCG CaMKIV is a CaM-dependent protein kinase and, as introduced earlier, is found predominately in cells of nervous and haematopoietic systems compared with the other CaMKs. A previous study also showed that CaMKIV was involved in murine HSC maintenance [17] . We were concerned whether CaMKIV was inactivated in iqcg morphants. As expected, whole-mount immunofluorescence data showed that the level of phosphorylated CaMKIV was markedly reduced in iqcg morphants compared with control embryos ( Fig. 1l ). To confirm that the inactivation of CaMKIV led to the depletion of HSC, we did rescue experiments. The WT and a series of CaMKIV mutant constructs were made, including constitutively active CaMKIV ( CACaMKIV ) with the autoinhibitory region deleted; dominant-negative DNCaMKIV (K58E) that diminished ATP binding at the catalytic site; and DNCaMKIV (T183A) that was a phosphorylation-defective mutant [26] , [27] , [28] ( Supplementary Fig. 2b ). The Flag-tagged WT CaMKIV as well as all the mutant constructs expressed comparatively in the HEK293T cells ( Supplementary Fig. 2c ). In the embryos co-injected with iqcg morpholino and mRNA for WT CaMKIV or CACaMKIV , the c-myb expression in the AGM was partially restored, although the rescue ratio of WT CaMKIV (32 in 51) being lower than CACaMKIV (29 in 39) ( Fig. 1m–p ). In contrast, the co-injections with DNCaMKIV (K58E) or DNCaMKIV (T183A) mRNA and iqcg morpholino were not able to rescue the c-myb expression ( Fig. 1q,r ). These results were also confirmed in the c-myb:eGFP transgenic line. As anticipated, both WT CaMKIV and CACaMKIV mRNA partially rescued the GFP + cell number in the CHT, whereas DNCaMKIV (K58E) or DNCaMKIV (T183A) mRNA did not ( Supplementary Fig. 2a ). To further confirm that CaMKIV acts downstream of Iqcg, we designed a camkIV -specific MO that was able to efficiently and specifically block the translation of the EGFP reporter that contains the sequence targeted by camkIV MO ( Supplementary Fig. 2d–f ). The results showed that camkIV morpholino knockdown phenocopied iqcg morphants in marker gene expression levels for HSC and differentiated haematopoietic cells ( Supplementary Fig. 2g–k ). These results suggested that CaMKIV acted as a downstream molecule of Iqcg in zebrafish haematopoiesis. Iqcg or camkIV knockdown impairs c-myb + cells proliferation We next assessed the impact of the reduction of iqcg or camkIV expression level on the cellular defects of c-myb + cells in the CHT. The phospho-histone 3 (pH3)-positive cells represent the mitotic cells in the M phase [29] . We checked the proliferation status of iqcg and camkIV morphants by using the staining of pH3. As shown in Fig. 3 and Supplementary Table 1 , double staining revealed that the percentage of pH3 + / c-myb + cells in the CHT was significantly decreased from 6.71% in controls to 1.69% in iqcg morphants ( P =0.007, n =9) and 1.44% in camkIV morphants ( P =0.009, n =12), indicating that depletion of HSC in iqcg and camkIV morphants may both be because of defective proliferation. As expected, CACaMKIV could significantly rescue the proliferation defect of c-myb + cells ( P =0.0138, n =12), whereas WT CaMKIV could also partially rescue this defect ( P =0.0522, n =16). 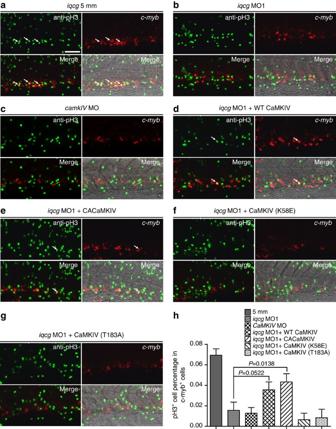Figure 3: Examination of cellular defects iniqcg-deficientc-myb+cells. (a–g) Double staining ofc-myband pH3 in the CHT of controls (a),iqcgmorphants (b) and camkIV morphants (c). Rescue experiments within vitrosynthesized WT CaMKIV (d), CACaMKIV (e), DNCaMKIV (K58E) (f) or DNCaMKIV (T183A) (g) mRNAs. Arrows indicatec-myband pH3 double-positive cells. Scale bar, 50 μm. (h) Histogram represents the percentage of pH3+/c-myb+cells in each experimental group. At least three independent experiments were performed. Results are expressed as means±s.e.m. GraphPad Prism software was used for statistical analysis. Student’st-test was used for determining the significance of the results.P<0.05 was considered statistically significant. Figure 3: Examination of cellular defects in iqcg -deficient c-myb + cells. ( a – g ) Double staining of c-myb and pH3 in the CHT of controls ( a ), iqcg morphants ( b ) and camkIV morphants ( c ). Rescue experiments with in vitro synthesized WT CaMKIV ( d ), CACaMKIV ( e ), DNCaMKIV (K58E) ( f ) or DNCaMKIV (T183A) ( g ) mRNAs. Arrows indicate c-myb and pH3 double-positive cells. Scale bar, 50 μm. ( h ) Histogram represents the percentage of pH3 + / c-myb + cells in each experimental group. At least three independent experiments were performed. Results are expressed as means±s.e.m. GraphPad Prism software was used for statistical analysis. Student’s t -test was used for determining the significance of the results. P <0.05 was considered statistically significant. Full size image IQCG–CaM structures reveal distinct CaM-binding footprints In an effort to elucidate the detailed mechanisms by which IQCG acts upstream of CaMKIV via binding CaM, we determined crystal structures of the IQCG IQ motif in complex with Ca 2+ -free and Ca 2+ -bound CaM to the resolutions of 1.5 and 2.1 Å, respectively ( Table 1 and Fig. 4a,b ). Table 1 Data collection and refinement statistics. 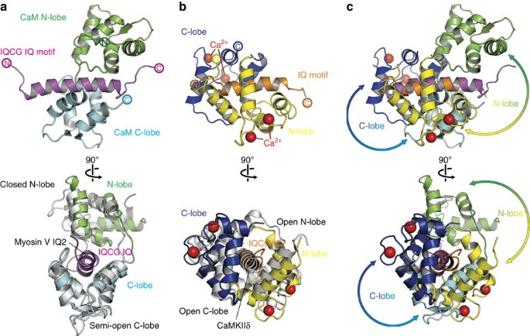Figure 4: Ca2+-induced conformational changes of CaM determine its distinct interactions with IQCG. (a) Cartoon representation of the Ca2+-free CaM (N-lobe coloured in green, whereas C-lobe in cyan) in complex with IQCG IQ motif (in magenta) compared with its complex with IQ2 from myosin V (in white; lower panel). (b) Ca2+-bound CaM (N-lobe in yellow, whereas C-lobe in blue) in complex with IQCG (in orange) compared with its complex with CaMKIIδ (in white; lower panel). Ca2+ions are shown as red spheres. (c) Superposition of the Ca2+-bound CaM–IQCG complex on the Ca2+-free counterpart based on the IQ motif (residues 400–410) of IQCG. Note that the conformations of each CaM lobe as well as the positions of the lobes undergo large changes as a result of Ca2+binding. Full size table Figure 4: Ca 2+ -induced conformational changes of CaM determine its distinct interactions with IQCG. ( a ) Cartoon representation of the Ca 2+ -free CaM (N-lobe coloured in green, whereas C-lobe in cyan) in complex with IQCG IQ motif (in magenta) compared with its complex with IQ2 from myosin V (in white; lower panel). ( b ) Ca 2+ -bound CaM (N-lobe in yellow, whereas C-lobe in blue) in complex with IQCG (in orange) compared with its complex with CaMKIIδ (in white; lower panel). Ca 2+ ions are shown as red spheres. ( c ) Superposition of the Ca 2+ -bound CaM–IQCG complex on the Ca 2+ -free counterpart based on the IQ motif (residues 400–410) of IQCG. Note that the conformations of each CaM lobe as well as the positions of the lobes undergo large changes as a result of Ca 2+ binding. Full size image The Ca 2+ -free complex illustrates the recognition of an IQ motif by CaM, reminiscent of the myosin V–CaM complex [13] ( Fig. 4a and Supplementary Fig. 3a ). The C-lobe of CaM adopts a semi-open [13] conformation and exposes hydrophobic residues within the domain to interact tightly with the N-terminal sequence of the IQ motif (L[I]QxxxR), while the N-lobe assumes the closed [13] conformation and binds to the C-terminal region of the IQ motif (GxxxR) ( Fig. 4a ). Specifically, at the first part of the IQ motif, the apolar side chains of IQCG residues L400, W403 and W404 insert snugly into the hydrophobic cleft of the CaM C-lobe ( Fig. 5a and Supplementary Fig. 4a ) whereas the hydrophilic side chains of motif-defining Q401 and R405 critically coordinate a network of hydrogen bonds and salt bridges between the binding partners to stabilize the structure, especially a loop between the pair of EF hands of the C-lobe ( Fig. 5a ). Significantly, the alanine substitution of Q401 (or Q312 in zebrafish Iqcg), which is invariable in the IQ motif, abolished the binding between IQCG and CaM in our Co-IP assay ( Fig. 5c ). At the second half of the IQ motif, the hydrophobic CaM–IQCG interactions involving IQCG residues M408 and I409 were comparatively less pronounced ( Fig. 5a ), yet R410 at the end of the consensus IQ sequence motif forms multiple hydrogen bonds with the CaM N-lobe, again in the middle of the two halves of the lobe. Thus, the overall interface between the IQCG IQ motif and the Ca 2+ -free CaM features both hydrophobic and hydrophilic interactions, a character shared by many CaM–target recognitions ( Fig. 5a,b ). 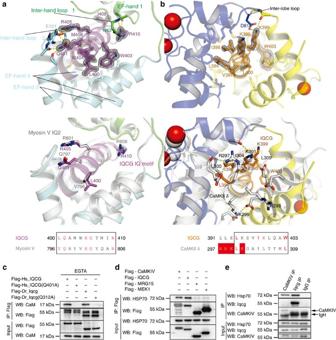Figure 5: Characteristics of the CaM–IQCG interfaces and ability of IQCG and CaMKIV to interact with HSP70. (a) IQCG uses a collection of both hydrophobic and hydrophilic residues (well-defined side chains as sticks in electron density map as grey mesh) to bind CaM in the Ca2+-free setting. The IQ motif-defining residues (coloured red in the lower panel) undertake almost identical conformations when compared with the CaM–myosin V IQ2 complex (middle panel). Dashed lines indicate salt bridges or hydrogen bonds. (b) A compromise in charge complementarity is evident at the interface between IQCG and Ca2+-bound CaM when compared with either the Ca2+-free complex (a) or a CaMKIIδ–CaM complex (middle panel). The colouring scheme is kept consistent withFig. 4and the superpositions were carried out based on the boxed sequences shown in the lower panels and so were those forFig. 4. The electron density is shown asσA-weighted 2Fo−Fcmap contoured at either 2σ(a) or 1.5σ(b). (c) A single-point mutated forms of IQCG, Hs_IQCG (Q401A) or Dr_Iqcg (Q312A) lost the ability to interact with CaM. (d) Ability of IQCG and CaMKIV to interact with HSP70, as determined by Co-IP experiments. Two irrelevant proteins, MRG15 and MEK1, are shown as negative controls. Anti-Flag M2 affinity gel was used for IP; an antibody to HSP70 or Flag was used for western blot (WB). (e) Ability of endogenic Iqcg and CaMKIV to interact with Hsp70. Co-IP experiments were performed using mouse testis lysate. Antibodies to CaMKIV, Iqcg and normal rabbit IgG were used for IP; antibodies to HSP70, Iqcg and CaMKIV were used for WB. Figure 5: Characteristics of the CaM–IQCG interfaces and ability of IQCG and CaMKIV to interact with HSP70. ( a ) IQCG uses a collection of both hydrophobic and hydrophilic residues (well-defined side chains as sticks in electron density map as grey mesh) to bind CaM in the Ca 2+ -free setting. The IQ motif-defining residues (coloured red in the lower panel) undertake almost identical conformations when compared with the CaM–myosin V IQ2 complex (middle panel). Dashed lines indicate salt bridges or hydrogen bonds. ( b ) A compromise in charge complementarity is evident at the interface between IQCG and Ca 2+ -bound CaM when compared with either the Ca 2+ -free complex ( a ) or a CaMKIIδ–CaM complex (middle panel). The colouring scheme is kept consistent with Fig. 4 and the superpositions were carried out based on the boxed sequences shown in the lower panels and so were those for Fig. 4 . The electron density is shown as σ A -weighted 2 F o − F c map contoured at either 2 σ ( a ) or 1.5 σ ( b ). ( c ) A single-point mutated forms of IQCG, Hs_IQCG (Q401A) or Dr_Iqcg (Q312A) lost the ability to interact with CaM. ( d ) Ability of IQCG and CaMKIV to interact with HSP70, as determined by Co-IP experiments. Two irrelevant proteins, MRG15 and MEK1, are shown as negative controls. Anti-Flag M2 affinity gel was used for IP; an antibody to HSP70 or Flag was used for western blot (WB). ( e ) Ability of endogenic Iqcg and CaMKIV to interact with Hsp70. Co-IP experiments were performed using mouse testis lysate. Antibodies to CaMKIV, Iqcg and normal rabbit IgG were used for IP; antibodies to HSP70, Iqcg and CaMKIV were used for WB. Full size image The Ca 2+ -bound CaM forms complex with the IQ motif on a distinct set of footprints, as revealed by the crystal structure ( Fig. 4b and Supplementary Fig. 3b ). L394 and W403 of the IQCG serve as the principal hydrophobic anchors to CaM, in a way similar to the CaMKIIδ autoinhibitory region [30] ( Fig. 5b and Supplementary Fig. 4b ). In this complex, although the contribution of the hydrophobic interactions involving L394, V397, I398, L400 and W403 from IQCG appears comparable to the Ca 2+ -free complex described above and other CaM–target complexes ( Fig. 5a,b ), the hydrophilic component of nanomolar affinity CaM–target recognitions is largely missing ( Fig. 5a,b ). Across the major binding site, only K399 provided noticeable hydrophilic interactions with CaM ( Fig. 5b ). This was not surprising as the primary sequence of the Ca 2+ -bound CaM-binding footprints on IQCG was less basic than typical Ca 2+ -dependent CaM-binding motifs [31] ( Fig. 5b , lower panel). In comparison, the Ca 2+ -bound CaM–CaMKIIδ complex [30] revealed the essential contribution of 4 basic residues from the CaMKIIδ autoinhibitory region to its interaction with CaM ( Fig. 5b , middle panel). Therefore, this Ca 2+ -bound complex demonstrated a non-canonical Ca 2+ -dependent CaM-binding sequence in the IQ domain of IQCG ( Fig. 5b ). The loss of critical hydrophilic interactions in the Ca 2+ -bound complex compared with the Ca 2+ -free version as well as other CaM–target complexes provided the structural basis for the apparently different binding affinities between IQCG and CaM in the presence or absence of Ca 2+ measured in our binding assays and data from previous study [30] . IQCG and CaMKIV could respectively interact with HSP70 Our results showed that IQCG positively regulated CaMKIV signalling in zebrafish haematopoiesis. It is well established that CaM activates CaMKIV by Ca 2+ -dependent sequestration of the kinase’s autoinhibitory domain [19] . Structural comparisons between our presented CaM–IQCG complexes and CaM–CaMK complexes would predict mutually exclusive binding of the peptides to CaM, which precludes a model in which IQCG binding to CaM directly helps with CaMKIV activation. Indeed, no direct interaction between IQCG and CaMKIV was observed using Co-IP in HEK293T cells ( Supplementary Fig. 5a ). We therefore hypothesized that IQCG may act as a reservoir for CaM when Ca 2+ level is low, and release CaM to activate CaMKIV when Ca 2+ level rises. A prediction from this hypothesis is that there might exist a molecular scaffold binding IQCG and CaMKIV. Immunofluorescence staining of HEK293T cells transiently transfected with plasmids expressing GFP–IQCG and Flag-tagged CaMKIV demonstrated that both proteins distributed in the cytoplasm ( Supplementary Fig. 5b ). To test the hypothesis, we tried to identify other proteins interacting with both IQCG and CaMKIV by Co-IP followed by mass spectrometric analysis. Two specific protein bands in the Flag–IQCG overexpressed sample were identified ( Supplementary Fig. 5c ). The upper band was heat-shock cognate 71 kDa protein that has also been named heat-shock 70 kDa protein 8 (Swiss-Prot Database accession number P11142 ). The lower band was identified as heat-shock 70 kDa protein 1 l (Swiss-Prot Database accession number P34931 ) ( Supplementary Fig. 5d ). Further binding assays demonstrated that both IQCG and CaMKIV precipitated HSP70 ( Fig. 5d ). In contrast, two irrelevant proteins MRG15 and MEK1 could not precipitate HSP70. To further confirm the interaction of endogenous IQCG and CaMKIV with HSP70, we performed Co-IP assay using mouse testis lysate where Iqcg was highly expressed, because there were more materials for experiments with mouse testis and we disposed quality antibodies only against murine Iqcg. Indeed, Hsp70 could be stained in the immunocomplexes captured by antibody to CaMKIV or Iqcg, but did not appear in the IgG-bound proteins ( Fig. 5e ). IQCG and HSP70 could cooperate in haematopoiesis To address the functional significance of interaction between Iqcg and Hsp70, we next carried out hsp70 knockdown assay in zebrafish using hsp70 morpholino as reported [32] , [33] . Western blot results showed that this hsp70 MO could efficiently knockdown Hsp70 protein expression ( Supplementary Fig. 5e ). In addition to a phenotype of affected blood circulation at the ca and cv, which could be related to the previously reported defect in embryonic vascularization [32] , the hsp70 morphants showed a partially reduced haematopoiesis in zebrafish, as evidenced by a reduced, c-myb expression level in the CHT at 3 d.p.f., a decreased staining of mpo at 36 h.p.f. and rag1 at 5 d.p.f., as well as a slightly reduced haemoglobin level ( Supplementary Fig. 5f–j ). Notably, in hsp70 morphants, whole-mount immunofluorescence assay revealed a decrease of phosphorylated CaMKIV level, suggesting that the partial defect of haematopoiesis at reduced Hsp70 level could be related to calcium signalling ( Supplementary Fig. 5k ). In addition, we tried to perform experiments with low doses of iqcg MO and hsp70 MO, which when used alone did not cause obvious phenotypes. Coinjection of these two MOs at low dose, in contrast, led to severe definitive haematopoietic defect in almost the similar way as did the standard dose of iqcg MO ( Supplementary Fig. 5l ). Therefore, Hsp70 may cooperate with Iqcg and participate in zebrafish definitive haematopoiesis. Calcium signalling participates in nearly all life processes from cellular to organism level. CaM is a ubiquitous calcium-binding protein, which is highly conserved between species. The amino-acid sequences of CaM proteins among human, mouse and zebrafish are completely identical. Many genes and encoded proteins are also evolutionarily conserved in calcium signalling pathway with CaM at the centre [15] . In the present study, we explored the function of a CaM-binding protein IQCG that was involved in the fusion with NUP98 in a patient with acute leukaemia. We found IQCG was critical for zebrafish definitive haematopoietic development, getting new insights into the regulation of haematopoiesis. Calcium signalling has a critical role in homeostasis of haematopoietic system. In mammals, HSCs within the bone marrow cavity reside close to the endosteal surfaces of bone, which have a high concentration of calcium ions [34] , [35] , [36] . HSCs respond to extracellular ionic calcium concentrations through the seven-pass transmembrane calcium-sensing receptor (CaR) [37] . The stimulation of CaR activates chemokine (C-X-C motif) receptor 4 (CXCR4) and integrin of HSCs, which contributes to engraftment. Owing to defective adhesion to collagen I, an extracellular matrix protein [38] , CaR −/− HSCs were highly defective in localizing anatomically to the endosteal niche. At the level of intracellular calcium-dependent cascades in haematopoietic cells, previous works focused on T lymphocytes. The elevation of intracellular calcium ion concentration activates calcium-dependent enzymes, such as calcinerin, CaMKIV and IKK. These proteins subsequently activate transcription factors, such as nuclear factor of activated T cells, cAMP-responsive element-binding protein and nuclear factor of kappa light polypeptide gene enhancer in B-cells [39] . It was reported that malignant T cells possessed elevated amounts of voltage-dependent Ca 2+ channels compared with normal T cells [40] . The elevation of cytosolic Ca 2 + level and subsequently activation of nuclear factor of activated T cells-mediated transcription in a Ca 2+ -dependent manner critically contributed to human T lymphotropic virus type 1 that caused T-cell leukaemia [41] . In HSCs, the importance of calcium signalling pathway was revealed by a study showing that CaMKIV was implicated in HSC maintenance [17] . In the present work, we found that in zebrafish, iqcg controlled definitive haematopoiesis through CaM-mediated calcium signalling and acted as an upstream molecule of CaMKIV. We therefore provide new evidence that calcium-dependent cascades are critical for proliferation of vertebrate HSC population. An intriguing feature of IQCG in regulating calcium signalling is to form complexes of distinct affinities with CaM in a cytoplasmic calcium concentration-dependent manner, as shown by Co-IP assay that IQCG could not precipitate Ca 2+ -bound CaM in cells. This observation has also gotten support from in vitro binding assays when Ca 2+ concentration was low, IQCG interacted with CaM tightly ( K D =5.07 nM); whereas in the presence of elevated Ca 2+ concentration, IQCG displayed a low binding strength with CaM ( K D =180 nM). This property could render Ca 2+ -bound CaM more likely to interact, in the cellular context, with proteins with higher binding potential, such as CaMKIV (previously reported binding constant with CaM 9 nM) [30] . Notably, we showed that HSP70 could form complex with both IQCG and CaMKIV. Based on these data, we propose a model in which a multi-component protein complex including HSP70 could harbour IQCG as a store of CaM to facilitate the regulation of the activity of CaMKIV ( Fig. 6 ). In other words, IQCG and CaMKIV may compete with each other in close vicinity for binding with CaM in a calcium concentration-dependent way. The chaperone machines have been reported to act as molecular scaffolds to regulate >200 signalling proteins, of which the most well-known protein is endothelial nitric oxide synthase [42] , [43] , [44] . The multi-chaperone machine can also stabilize steroid receptors by modulating ligand-binding clefts [44] . Here, we suggest that HSP70 might serve as a scaffold to bind both IQCG and CaMKIV, thereby facilitating the regulation of the activity of CaMKIV. This hypothesis was supported by our functional data showing cooperation between Iqcg and Hsp70 in maintaining the zebrafish haematopoiesis. 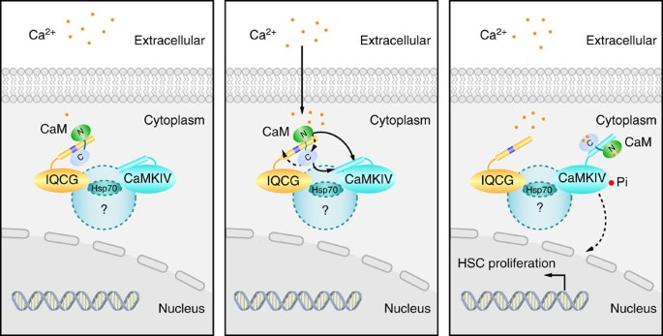Figure 6: Proposed mechanism of IQCG in calcium/CaM signalling. The cytoplasmic Ca2+level is low in resting cells and IQCG binds Ca2+-free CaM via the IQ motif (left panel). When specific signals trigger an increase of the cytoplasmic Ca2+level, the affinity between CaM and IQ motif decreases. As IQCG and CaMKIV are hypothetically bound by putatively scaffold proteins including HSP70 and other unknown molecules in the complex (a big circle of question mark depicted with dotted line), both lobes of CaM may subsequently bind CaMKIV (indicated by solid line) instead of reassociating to the new sites of IQCG (indicated by dotted line; middle panel). The binding of CaM activates CaMKIV and its downstream pathway, and promotes cell proliferation (right panel). Figure 6: Proposed mechanism of IQCG in calcium/CaM signalling. The cytoplasmic Ca 2+ level is low in resting cells and IQCG binds Ca 2+ -free CaM via the IQ motif (left panel). When specific signals trigger an increase of the cytoplasmic Ca 2+ level, the affinity between CaM and IQ motif decreases. As IQCG and CaMKIV are hypothetically bound by putatively scaffold proteins including HSP70 and other unknown molecules in the complex (a big circle of question mark depicted with dotted line), both lobes of CaM may subsequently bind CaMKIV (indicated by solid line) instead of reassociating to the new sites of IQCG (indicated by dotted line; middle panel). The binding of CaM activates CaMKIV and its downstream pathway, and promotes cell proliferation (right panel). Full size image Our structural biology study was in support of this model. Although CaM binds to the IQ motif of IQCG in the absence of Ca 2+ ; in the Ca 2+ -bound state, CaM lodges at a non-canonical Ca 2+ -dependent CaM-binding sequence on IQCG shifted around six residues towards N-terminal from the Ca 2+ -free interaction site. This cryptic Ca 2+ -dependent CaM-binding sequence appears to be less positively charged than typical Ca 2+ -dependent CaM-binding motifs [31] , and as such, the many hydrophilic interactions that putatively contribute to the high-affinity bindings of CaM to target helices are missing in the Ca 2+ -bound complex of CaM and IQCG, which likely leads to the drop in the affinity from the Ca 2+ -free state. Moreover, with respect to the IQCG IQ helix, both lobes of CaM bind IQCG at different sites in distinct orientations ( Fig. 4c ). We speculate that this would further facilitate the competitions by partners possessing higher affinities such as CaMKs [30] because both CaM lobes would dissociate from IQCG. Some investigations demonstrated that the free intracellular CaM concentration could be limiting [45] , [46] , [47] . It is therefore of physiological significance that IQCG releases CaM and activates downstream target proteins. Finally, it is worth pointing out that in NUP98–IQCG fusion, there was a dislocation, from cytoplasm into nucleus, of not only fusion protein but also IQCG, owing to the heterocomplex formation between the fusion as a result of t(3;11)(q29q13;p15)del(3)(q29) and the IQCG proteins generated by the WT gene on undisrupted allele [7] . CaM distributes both in the cytoplasm and nucleus during interphase [48] . CaMKII and CaMKIV, which are downstream protein kinases of CaM, are both relevant to cell proliferation. It was reported that nuclear CaMKII can enhance histone H3 phosphorylation (a mitotic marker) [49] . cAMP-responsive element-binding protein, a transcription factor that can be activated by nuclear CaMKIV, is also critical for the proliferation of primary HSCs or myeloid leukaemia cells [50] . So we may postulate that transfer of CaM by aberrantly located NUP98–IQCG/IQCG complex to the improper downstream proteins might deregulate cellular calcium signalling pathways in haematopoietic stem/progenitor cells and thus promote excessive cell growth and block differentiation, ultimately contributing to leukaemogenesis. In conclusion, our data illuminate the function of iqcg in zebrafish haematopoietic development by a combination of developmental biology analysis and research into functions and structures of the protein. We find that iqcg is required for zebrafish definitive HSC proliferation. Furthermore, we show that IQCG binds to CaM and acts as a regulator of calcium signalling upstream of CaMKIV. These results also shed light on the pathogenesis of acute leukaemia with NUP98–IQCG fusion. Zebrafish strains The zebrafish facility and zebrafish study were approved by the Institutional Review Board of the Institute of Health Sciences, Shanghai Institutes of Biological Sciences, Chinese Academy of Sciences (Shanghai, China). Zebrafish stocks were maintained at 28.5 °C under standard aquaculture conditions. Embryos were staged by hours or days post fertilization (h.p.f. or d.p.f.) as described [51] . The Tg(c-myb:eGFP) transgenic zebrafish lines were the generous gifts from Prof. Leonard Zon’s lab. Cloning and plasmid construction The Zebrafish iqcg gene was identified based on homology to human IQCG. Full-length coding sequence for iqcg was obtained by reverse transcription (RT)–PCR and then cloned into pCS2+ (Addgene). WT CaMKIV, CACaMKIV, DNCaMKIV (K58E) and DNCaMKIV (T183A) were Flag tagged and cloned into pCS2+. cDNA Hs_IQCG, Hs_ΔIQCG, Dr_Iqcg, Dr_ΔIqcg and CaMKIV were amplified by PCR and cloned into pFlag-CMV4 (Sigma) or pEGFP-C1 (Clontech) vectors. Hs_IQCG (Q401A) and Dr_Iqcg (Q312A) were constructed by QuikChange Site-Directed Mutagenesis Kit (Agilent). Human CaM was cloned into RSFDuet-1 (Novagen). Human IQCG IQ motifs (residues 389–423 for Ca 2+ -free complex crystallization and SPR, residues 376–435 for Ca 2+ -bound complex crystallization) were cloned into the pGEX-6P-1 (GE Healthcare) expression vector. The primer sequences are presented in Supplementary Table 2 . Morpholino, mRNA synthesis and microinjection MOs were purchased from Gene Tools: iqcg MO1: 5′-TCCTCCACGGACATCATACTGCTAA-3′; iqcg MO2: 5′ CTAAACAAAGAGGCAAATCAGCCGT-3′; iqcg 5-mismatch MO: 5′-TCCTCgACgGAgATCATAgTcCTAA-3′; camkIV MO: 5′-CATTGTCACTTTCAGCATCTCCAGC-3′; hsp70 MO: TAGCGATTCCTTTTGGAGAAGACAT. Capped mRNAs were transcribed with mMESSAGE mMACHINE Kit (Ambion). For all the microinjection experiments, a volume of 2 nl was injected into one-cell stage embryos. For Supplementary Fig. S3I , the injection doses have been labelled; for other experiments, the injection doses per embryo were iqcg MO1, 6 ng; iqcg MO2, 6 ng; iqcg 5-mismatch MO, 6 ng; camkIV MO, 8 ng; and hsp 70 MO, 10 ng. In the case of rescue experiments, morpholino plus 100 pg mRNA were injected. Whole-mount mRNA in situ hybridization WISH was performed as reported [52] . Embryos were fixed in 4% paraformaldehyde at the indicated stages and further dehydrated using methanol. After rehydrated, embryos were digested by Proteinase K (Calbiochem) and fixed again. Then the embryos were prehybridized at 68 °C with HYB– buffer: 50% formamide, 5 × SSC, 0.1% Tween-20, 9.2 mM citric acid, pH 6.0, and further hybridized with 1 ng μl −1 -specific RNA probe in HYB+ buffer: 50% formamide, 5 × SSC, 0.1% Tween-20, 9.2 mM citric acid, pH 6.0, 500 μg ml −1 yeast tRNA and 50 μg ml −1 heparin. Antisense RNA probes were generated using digoxigenin-11-uridine 5_-triphosphate (Roche Applied Science). These probes were detected with alkaline phosphatase-conjugated antibodies (1:5,000; Roche Applied Science) using the substrates 5-bromo-4-chloro-3-indolyl phosphate/nitro blue tetrazolium (purple colour; Vector Laboratories, Burlingame, CA, USA). After staining, embryos were mounted in 4% methylcellulose and captured under the Nikon SMZ1500 stereomicroscope equipped with a Nikon DXM1200F digital camera and ACT-1 software. O-dianisidine stain Embryos at 4.5 d.p.f. were stained for 15 min in the dark in O-dianisidine (0.6 mg ml −1 ), 0.01 M sodium acetate (pH 4.5), 0.6% hydrogen peroxide and 40% (v/v) ethanol. Stained embryos were washed twice with PBS plus 1% Tween-20, and then were fixed in 4% paraformaldehyde for 1 h. Immunofluorescence The fixed embryos were dehydrated with methanol and kept at −20 °C overnight. After rehydration, the embryos were treated with Proteinase K (40 μg ml −1 ) for 30 min at 30 °C and re-fixed in 4% paraformaldehyde for 20 min. Following washing with PBST (0.1% Tween in PBS), the embryos were permeabilized in a solution containing 0.1% Triton X-100+0.1% sodium citrate in PBS for 1 h at room temperature (RT), rinsed with PBST and then blocked in PBST with 10% fetal bovine serum (FBS) for 1 h. Finally, the embryos were stained with anti-p-CaMKIV (1:100; Santa Cruz) at 4 °C overnight. After removing the primary antibody, the embryos were washed with PBST and finally incubated with Alexa Fluor 488-labelled goat anti-rabbit IgG antibody (1:200; Invitrogen). Double staining of c-myb RNA and pH3 protein Double staining of c-myb RNA and pH3 was performed as Du et al . described [53] . To detect c-myb RNA and mitosis marker pH3 simultaneously, embryos were first hybridized with the DIG-labelled antisense cmyb RNA probe. After washing and blocking, the embryos were incubated at 4 °C overnight with a peroxidase-conjugated anti-DIG antibody (1:500; Roche) and stained with Alexa Fluor Cy3-conjugated tyramide as substrate (PerkinElmer) according to the manufacturer’s instructions. After three 20-min washes with PBST at RT, the embryos were soaked in incubating buffer (PBS with 0.1% Triton X-100, 1% bovine serum albumin and 1% DMSO (dimethyl sulfoxide)) plus 2% lamb serum for 1 h at RT and then incubated with primary antibody anti-pH3 (ser10; 1:500; Santa Cruz Biotechnology) at 4 °C overnight. After removing the primary antibody, the embryos were washed with incubating buffer and finally incubated with fluorescein isothiocyanate (FITC)-labelled goat anti-rabbit IgG antibody (1:500; Molecular Probes). Images were taken using a Leica TCS SP5 confocal microscope. Cell culture, transfection, IP and western blot For IP experiments, we used HEK293T cell line or mouse testis. For HEK293T cells from ATCC, 10 μg Flag-tagged plasmids were transfected in 1.5 × 10 6 HEK293T cells using Superfect (Qiagen). After 48 h, the cells were lysed with 0.5 ml of lysis buffer (50 mM Tris HCl, pH 7.4, with 150 mM NaCl, 1% NP40 and 1 mM EGTA or 1 mM CaCl 2 supplemented with protease inhibitor cocktail). The immunocomplex was captured by incubating with anti-Flag M2 affinity gel (Sigma). Western blot was performed with anti-Flag (Sigma), anti-CaM (Millipore) or anti-HSP70 (BD Biosciences). For mouse testis, we lysed testis with lysis buffer. Antibodies (5 μg) to CaMKIV (Cell Signaling Technology) or Iqcg (against murine Iqcg amino acids 241–419, generated and purified by our lab), or normal rabbit IgG (Santa Cruz) were incubated with nProtein A Sepharose 4 Fast Flow (GE Healthcare) for 4 h, and then incubated with testis lysates overnight. For western blot analysis, an antibody to native rabbit IgG was used as second antibody for staining Iqcg, because mouse Iqcg has a similar molecular weight as IgG heavy chain. The original photos of western blots are shown in Supplementary Fig. 6 . Silver stain and mass spectrometry pFlag-CMV4 or Flag-tagged Hs_IQCG was transfected in HEK293T cells. Methods of transfection, cell lysis and IP were shown as above. Lysis buffer is Ca 2+ chelated. Bound proteins were analysed by SDS–PAGE and silver staining. Specific bands were excised and the protein sequences were determined using MALDI-TOF-TOF4700 mass spectrometer (ABI). Protein expression and purification All proteins were expressed in Escherichia coli BL21 (DE3). Cells were grown for 16 h after induction by 0.2 mM isopropyl-β-D-thiogalactopyranoside (IPTG) at 16 °C and harvested, and the pellet was lysed by sonication in lysis buffer (PBS containing 1 mM EDTA). The CaM–IQ complex was obtained by coexpression. All proteins with GST tag were purified by chromatography using glutathione Sepharose (GE Healthcare). The GST tag was cleaved by PreScission protease overnight at 4 °C and the protein with a five amino-acid tag at the N-terminal (-GPLGS-) was then eluted with lysis buffer. CaM was purified using Q-Sepharose chromatography with buffer A (10 mM HEPES, pH 7.5, 10 mM NaCl and 1 mM EDTA) and eluted with a linear gradient to 50% buffer B (10 mM HEPES, pH 7.5, 1 M NaCl and 1 mM EDTA). All the proteins were further polished by gel filtration using a Superdex 75 column (GE Healthcare) with buffer A or buffer C (10 mM HEPES, pH 7.5, 10 mM NaCl and 1 mM CaCl 2 ). Analysis of IQCG/CaM-binding kinetics using SPR Using a BIAcore 3000 SPR system, we analysed the binding of IQCG IQ motif (residues 389–423) to GST-CaM that had been immobilized on the surface of a CM5 sensor chip by amine coupling in absence and presence of Ca 2+ . Purified GST-CaM proteins were immobilized on CM5 sensor chips to final resonance values of ~1,000 response unit (RU). The concentrations of IQCG IQ motif were 8.4–50 nM for Ca 2+ -free, and 20–320 nM for Ca 2+ -supplemented condition. Various concentrations of analytes in HBS-P (10 mM HEPES, 150 mM NaCl, 0.005% surfactant P20, pH 7.4) containing 1 mM CaCl 2 or 3 mM EDTA were injected for 2 or 3 min (20 or 15 μl min −1 , respectively). 2-Mercaptoethanol was added to the running buffer at 0.1%. Each series of experiments was performed in duplicate. The sensor chips were regenerated by a 10-s injection of 50 mM NaOH. The sensorgrams were analysed using BIAevaluation software (version 3.1; BIAcore). All of the binding curves were collected by subtraction of reference flow cells. Large spikes at the beginning and the end of an injection are because of a difference in the refractive indices of the buffer alone and the buffer containing an analyte protein. The model used was the 1:1 Langmuir-binding interaction model. The association rate constant, K a , and the dissociation rate constant, K d , were determined by global fitting of the curves. The dissociation constant was determined by K D = K d / K a . The mean values of the rate constants and the dissociation constants were obtained from duplicate experiments for each concentration. Crystallization and data collection The purified proteins were concentrated to 20 mg ml −1 in buffer A (for Ca 2+ -free complex) or buffer C (Ca 2+ -bound complex) using a 10-K Filtron ultrafiltration membrane. Proteins were crystallized by vapour diffusion at 4 °C in a hanging drop format. The two CaM–IQ complexes were crystallized in the same condition, and the drop contained equal volumes of 20 mg ml −1 protein and the reservoir solution (1.6 M ammonium sulphate and 1 M lithium sulphate). Before collections, crystals were transferred and soaked into 88% saturated lithium sulphate for 15 s and then flash frozen to 83 K. Diffraction data were collected at Beamline 17U synchrotron, Shanghai Synchrotron Radiation Facility (SSRF, 17U). Structure determination and refinement X-ray diffraction data were processed using the HKL2000 package [54] . The Ca 2+ -bound structure was solved by molecular replacement in the programme Phaser [55] using the structure of CaM (Protein Data Bank accession code 3EWT ; chain A) as a search model. The Ca 2+ -free structure was solved by molecular replacement in the programme Phaser using the structure of CaM (N-lobe and C-lobe as the search models successively) from its complex with myosin V [13] (Protein Data Bank accession code 2IX7 ; chain A). With CaM placed, the electron density for the IQCG helix became immediately apparent in both complexes, which allowed automatic building by the programme ARP/wARP [56] . Clearly, there is one CaM–IQCG complex per asymmetric unit in both cases. The structures were then iteratively built manually in Coot [57] , refined (with riding hydrogens in the case of the Ca 2+ -free complex) in Phenix [58] , and validated with MolProbity [59] . The Ramachandran plots of both complex structures show 99.4% and 0% of their residues to be in the favoured and the disallowed regions, respectively. Structural figures were generated using PyMOL (Schrödinger) and organized in CorelDRAW (Corel) [60] . Statistical analysis Results are expressed as means±s.e.m. GraphPad Prism software was used for statistical analysis. Student’s t -test was used for determining the significance of the results. P <0.05 was considered statistically significant unless otherwise stated. How to cite this article: Chen, L.-T. et al . Functional and molecular features of the calmodulin-interacting protein IQCG required for haematopoiesis in zebrafish. Nat. Commun. 5:3811 doi: 10.1038/ncomms4811 (2014). Accession codes: Coordinates and structure factors for the crystal structures of CaM–IQCG complexes have been deposited in the Protein Data Bank under accession codes 4LZX for the Ca 2+ -free and 4M1L for the Ca 2+ -bound states, respectively.